Carrier separation and transport in perovskite solar cells studied by nanometre-scale profiling of electrical potential Organometal–halide perovskite solar cells have greatly improved in just a few years to a power conversion efficiency exceeding 20%. This technology shows unprecedented promise for terawatt-scale deployment of solar energy because of its low-cost, solution-based processing and earth-abundant materials. We have studied charge separation and transport in perovskite solar cells—which are the fundamental mechanisms of device operation and critical factors for power output—by determining the junction structure across the device using the nanoelectrical characterization technique of Kelvin probe force microscopy. The distribution of electrical potential across both planar and porous devices demonstrates p–n junction structure at the TiO 2 /perovskite interfaces and minority-carrier diffusion/drift operation of the devices, rather than the operation mechanism of either an excitonic cell or a p-i-n structure. Combining the potential profiling results with solar cell performance parameters measured on optimized and thickened devices, we find that carrier mobility is a main factor that needs to be improved for further gains in efficiency of the perovskite solar cells. A new emerging solar conversion technology, the organic–inorganic hybrid lead–halide perovskite (PS) solar cell, has attracted tremendous interest because of its combined advantages of high conversion efficiency, low-cost processing and the use of earth-abundant materials, which are critical factors for large-scale deployment of solar energy. The solar–electrical conversion efficiency of PS solar cells has been greatly improved to >20% in a few years [1] , [2] . In contrast, it took more than two decades of research and development to reach similar conversion efficiencies for first-generation crystalline silicon and second-generation inorganic thin-film solar cells [3] , which are the main conversion technologies in the solar industry today. The PS material has organic–inorganic hybrid characteristics in many aspects of material science and device physics. It has a well-defined crystalline structure and energy bandgap, similar to the traditional inorganic polycrystalline photovoltaic (PV) materials such as CdTe and Cu(In,Ga)Se 2 (CIGS). However, unlike the inorganic materials that usually require expensive vacuum processing to produce high-quality materials, the PS material crystalizes easily from solution phase. This enables utilization of inexpensive processing such as spin-coating and printing, which has been employed for producing organic solar cells but with their current record efficiencies still below 13% despite great research effort [4] . The hybrid characteristics are also manifested in the fundamental device structure. The design of a solar cell structure is decided primarily by the optical, electronic and electrical properties of the light-absorbing material, and it requires the optimization of the excitation, separation and transport of charge carriers. An inorganic thin-film cell is usually designed as either a planar p–n or a p–i–n junction [5] , depending on the minority-carrier diffusion length and doping concentration in the absorber. An organic cell is often designed in a bulk heterointerface structure [5] , because of the significant binding energy of excitons compared with the thermal energy at room temperature. The excitons, with short exciton diffusion lengths, need interfaces in close proximity to separate into free carriers. These device structures are usually highly material dependent; high-performance devices cannot usually be achieved in alternative structures for a particular absorber material. However, high-performance PS solar cells can be made in both planar and bulk heterointerface structures [6] , [7] . There is debate among the community as to which device structure is the most robust, thus a deeper understanding of the electrostatic potential within the device can guide device optimization. The PS cells with planar structure have reached efficiencies greater than 15–17% (ref. 8 ). Interestingly, the current record PS device has a combined structure of a mesoporous-PS layer at the bottom (in contact with the compact TiO 2 layer) followed by a planar PS-capping layer underneath the hole-transport layer (HTL) [2] . These characteristics of the PS cells are significantly different from both the traditional inorganic thin-film cells (for example, CdTe) and organic cells (for example, P3HT/PCBM) [5] . Two critical questions arise about this anomalous material: (1) are the photoexcited states bounded excitons or free-mobile electrons/holes? (2) Is transport of the carriers in this material diffusion-dominated or does it have to be field-assisted (drift)? Understanding these fundamental material properties is important for designing device structure and improving its performance. However, although the device efficiency has surpassed 20%, which is comparable to state-of-the-art crystalline Si and polycrystalline thin-film solar cells [4] , understanding the fundamental device operation mechanisms is still in its infancy [9] , [10] , [11] , [12] , [13] . First, there is paucity of characterization studies, as compared with the large numbers of publications for other materials that have been developed for decades. Second, because the device research and development is still at an early stage, variations in devices and materials induced by processing imperfections make it difficult to properly identify intrinsic material properties. For example, the superior devices of CH 3 NH 3 PbI 3− x Cl x over CH 3 NH 3 PbI 3, and the structure of a mesoporous Al 2 O 3 scaffold over the planar structure, are mainly due to the processing-dependent PS film quality, rather than the intrinsic material properties. CH 3 NH 3 PbI 3− x Cl x and CH 3 NH 3 PbI 3 devices, either in a planar or scaffold structure, have both reached similar high performance with high-quality PS films [2] . Third, some artefacts and modification of the devices during characterization can easily complicate the results and interpretations, which is expected to occur especially for the PS material with relatively unstable mechanical, structural and optoelectronic properties. As a result, the PS material may change significantly during characterization studies due to interactions with a probe, beam, electric current and/or field. In this report, we address the important questions mentioned above by profiling the electric potential (or field) across the devices using Kelvin probe force microscopy (KPFM) [14] , [15] , [16] , and by combining the potential data with the examination of device performance changes as a function of the PS absorber layer thickness. The high-performance devices we have studied ensure that the results are representative of the materials and device physics associated with efficient PV operation. The KPFM probe does not electrically interact with the materials, because the electric field between the probe and sample is constantly nullified during the measurement [10] , [11] . KPFM has been used previously to characterize the potentials at grain boundaries (GBs) from the top surface of the PS films [17] , [18] as well as to study the potential distribution across the device stack by monitoring the potentials in the cross-section of PS solar cells [11] , [12] , [17] . For the latter studies, inconsistent results of the junction types were reported with limited device structures [11] , [12] . These cross-sectional KPFM studies were based on profiling across devices without changing the bias voltage, which cannot exclude the influence of surface charges (defects) created on the cross-sectional surface during sample cleaving and preparation. Moreover, local facets of grains on the cleaved cross-sectional surface can have uncontrollable defects/charges in comparison with the top surface of the PS film [17] , [18] . To avoid the influence of surface charges on the measurement and interpretation, we have developed a procedure to measure surface potential changes by applying a series of bias voltages. In this condition, the change of the surface potential is about the same as the potential change in the bulk and the effect of surface charge can be excluded [19] , [20] , [21] , [22] . Our potential profiling results on both planar and porous devices with varying PS film thickness (from about 240 to 1,000 nm) show convincingly that the device physics of the PS solar cells resembles that of the traditional inorganic polycrystalline PV devices [5] , where a p–n junction is located at the TiO 2 /PS interface and free-carrier concentration is on the order of 10 16 –10 17 cm −3 . However, unlike the polycrystalline cells, the diffusion length of minority carriers for thicker devices is likely shorter, which is presumably associated with poor carrier transport across the thick PS layer. KPFM characterization Based on the atomic force microscopy (AFM) technique, KPFM measures contact potential difference between the probe and the surface of a solid-state sample by constantly probing and nullifying the Coulomb force between the probe and the sample. It maps the electrostatic potential of the sample surface with spatial and energy resolutions of 30–50 nm and ∼ 10 meV, respectively [14] , [15] , [16] . 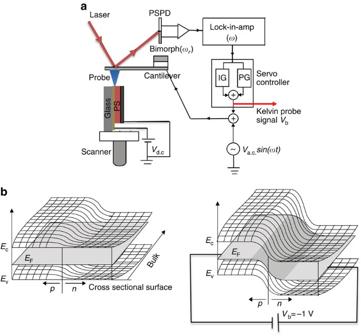Figure 1: Schematics of KPFM and identification of bulkp–njunction by surface potential. (a) KPFM set-up. (b) Left panel: potential configuration around ap–njunction without aVbapplied to the device, and right panel: potential configuration with a reverseVbapplied to the device. The surface potential around the junction is flattened by surface band-bending, as shown in the left panel. The right panel illustrates ap–njunction exposure onto the surface potential by applying aVbto the device. Figure 1a shows a schematic diagram of the set-up. To profile the potential across the device, we cleaved the device to expose the cross-section. The cross-sectional surface should not be further processed (such as by being polished), as long as effective AFM and KPFM imaging can be adequately performed [19] , [20] . This fact is important for cross-sectional KPFM, because the KPFM measurements are highly surface-sensitive and any modification of the surface region may induce significant artefacts. For example, a treatment, which does not even significantly change the device current–voltage (I–V) output, may significantly change the cross-sectional surface region, because the change in the surface region may have only a minor effect on the overall device output. Our KPFM is set in a glove box with H 2 O and O 2 concentrations of <0.1 p.p.m., which helps mitigate the effect of humidity and oxidation that might complicate the analysis. Figure 1: Schematics of KPFM and identification of bulk p – n junction by surface potential. ( a ) KPFM set-up. ( b ) Left panel: potential configuration around a p–n junction without a V b applied to the device, and right panel: potential configuration with a reverse V b applied to the device. The surface potential around the junction is flattened by surface band-bending, as shown in the left panel. The right panel illustrates a p–n junction exposure onto the surface potential by applying a V b to the device. Full size image The surface potential is determined by charges trapped on the cross-sectional surface and in the near-surface region. Any charges deeper than a screening length (in the range of hundreds of nanometres for most PV materials) should have negligible effect on the surface potential. In this characterization study, our primary goal is to profile the electrical potential in the bulk of the device to extract information about carrier separation and transport. Therefore, we must obtain information about the bulk property using a surface-potential measurement. To achieve this goal, we developed a procedure to measure the change in the surface potential induced by applying a bias voltage ( V b ) to a working device [19] , [20] , [21] , [22] . The change in surface potential should be about the same as the potential change in the bulk, provided V b is sufficiently small (such as 1–2 V). In other words, we can obtain the potential change in the bulk by measuring the change in surface potential, because the configuration of surface charges trapped at the localized surface states should not change significantly with such a small V b . Figure 1b schematically illustrates that the built-in potential of a p–n junction can be flattened by the surface band-bending (or surface charges), such that the bulk built-in potential ( V bi ) of the junction does not appear properly on the surface (left panel). The junction location can be produced on the surface potential by applying a V b to the junction (right panel). We have demonstrated this identification of junction location on many inorganic solar cells with the location accuracy of a few tens of nanometres [19] , [20] , [21] , [22] . Thin planar devices We first discuss the potential profiling results from a planar device with the PS thickness of ∼ 240 nm. The I–V curve and solar cell performance parameters are shown in Fig. 2 and Table 1 , respectively. The device subjected to the potential profiling has an efficiency of 16.1%. The good device performance ensures that our potential profiling results are relevant to the operation of an efficient solar cell device and not dominated by other variables in the device processing or resulting from poorly performing contacts. Figure 3b,c shows an AFM topographic and the corresponding KPFM potential images, respectively. 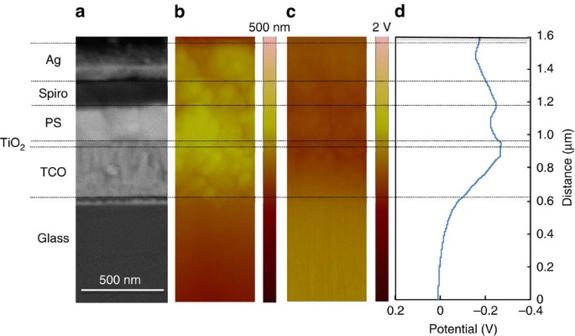Figure 3: Layered structure and potential imaging of the optimized planar device. (a) SEM image; (b) AFM and (c) the corresponding KPFM images taken on the cross-sectional surface of the 240-nm planar PS device. (d) Potential profile averaged fromcalong the lateral direction. The images were taken underVb=0 V. Scale bars of the AFM and KPFM indicate relative scales of the surface corrugation and surface potential. The positions of the layers are indicated on the left of the figure, which are identified from the SEM image. The scale bars are set much larger than the actual data range to best display the image contrasts. Figure 3d is a potential profile averaged from 64 scan lines of the potential image along the lateral direction. This average procedure is necessary to obtain reliable potential data, because it mitigates any local artefacts that may occur locally on the cross-sectional surface, and significantly improves the signal/noise ratio of the potential data. The thickness nonuniformity of the devices is small; the average over 500–800 nm scan size (64 lines) blurs the interfaces on the order of 10 nm, which is compatible with the KPFM resolution. To identify the device layers, we took scanning electron microscopy (SEM) images of the cross-section ( Fig. 3a ), which align well with the AFM and KPFM images. The secondary electron density is determined by many factors such as chemistry, workfunction, doping and morphology, and thus provides sufficient contrast between the various material layers in the PS device. 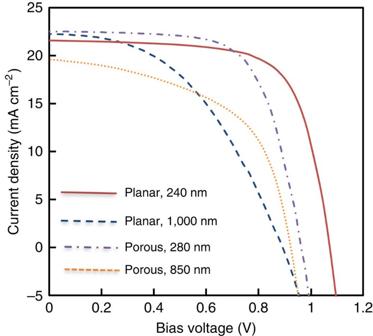The length scales of both AFM and SEM were calibrated within 2% and the misalignment of the layer locations between AFM and SEM is within ±20 nm, which is also compatible with the KPFM resolution. Figure 2:J–Vcurves of the four PS solar cell devices subjected to the potential profiling study. The measurement was carried out under one-sun illumination in a solar simulator. Figure 2: J–V curves of the four PS solar cell devices subjected to the potential profiling study. The measurement was carried out under one-sun illumination in a solar simulator. Full size image Table 1 Photovoltaic performance parameters and thickness of the solar cells. Full size table Figure 3: Layered structure and potential imaging of the optimized planar device. ( a ) SEM image; ( b ) AFM and ( c ) the corresponding KPFM images taken on the cross-sectional surface of the 240-nm planar PS device. ( d ) Potential profile averaged from c along the lateral direction. The images were taken under V b =0 V. Scale bars of the AFM and KPFM indicate relative scales of the surface corrugation and surface potential. The positions of the layers are indicated on the left of the figure, which are identified from the SEM image. Full size image Ideally, the potential image taken under V b =0 should reflect the workfunction contrast between the layer materials if the charges on the cross-sectional surface are uniform or the surface is not charged. However, it is clear from the measured potential profile that the potential is highly nonuniform within a single layer, and there is little contrast between the layers. In fact, this potential contrast changes from area to area, and it is not independent on the surface morphology. As noted earlier, the surface potential contrast is dominated by the nonuniformly distributed surface charges, which is unavoidable because of the particular local surface structure/configuration [19] , [20] , [21] , [22] . The surface-potential distribution should depend on the local surface charge-trapping. The GB potential contrast was not reliably observed on the cross-sectional surface, because the surface charge distribution depends on local cross-section cleaving. Local facets of grains can have many uncontrollable defects/charges, which are different from the potential mapping on the plane-view surface of the film [17] , [18] . To determine the bulk potential profile from the surface measurement, we apply a series of bias voltages V b s to the device, and image the surface potential under each V b (see Supplementary Fig. 1 ). The potential images with the various V b s must be taken on the same surface area, and the roughness of the area should be sufficiently small to ensure that there are no significant artefacts. Also, we must take an average over a certain distance (at least a few hundred nanometres) in the device lateral direction to ensure a representative potential profiling across the device; one line profile or the average from repeated measurements along the same line or from multiple lines over a relatively short distance (for example, a few nanometres) may not be representative [19] , [20] , [21] , [22] . 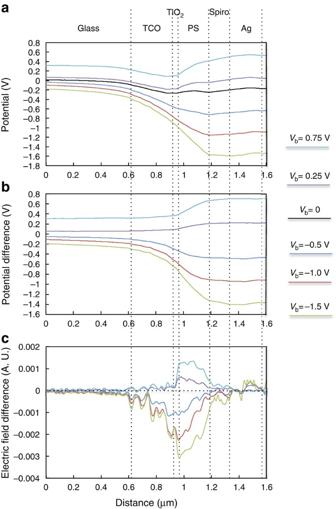Figure 4: Electrical potential and field profiling results on the optimized planar device. (a) Potential profiles taken on the 240-nm device under variousVbs. (b) Differences or changes between the potentials at the variousVbs andVb=0. (c) Change in the electric field byVbs. The potential profiles inaare averaged from the potential images along the device lateral direction. The potential changes inbare obtained by subtracting the potential underVb=0 from the potentials under the variousVbs. The profiles of the electric field difference incare deduced by taking a derivative of the potential differences inb. Layer positions are indicated on top of the figure, which are identified from the SEM image shown inFig. 3a. The potential change inband the field change incconcentrate around the TiO2/PS interface, and decrease towards the HTL, which is consistent with ap–njunction at the interface. Figure 4a shows the potential profiles averaged from the potential images ( Supplementary Fig. 1 ) with varying V b from −1.5 V (reverse) to +0.75 V (forward). Figure 4b shows the potential changes from the V b =0 case. This is obtained by simply subtracting the V b =0 potential from those obtained at various V b s to eliminate the effect of static surface charge. Further, we took the first derivative of the potential difference to obtain the V b -induced electric field distribution, as shown in Fig. 4c . From the potential and field results, one observes that the potential drop or the electric field occurs over the n -type layers of transparent conducting oxide (TCO) and TiO 2 , and the PS absorber layer. The electric field maximum is located at the TiO 2 /PS interface, and the field decreases towards the HTL side. This potential/field picture indicates that the PS and the TiO 2 /TCO layers form a p–n junction. This is different from both an excitonic cell and an n–i–p junction of free carriers, because in both cases one would expect a relatively uniform electric field across the absorber layer [5] . It is worth noting that for a planar device without the HTL (spiro-OMeTAD), the KPFM profile is the same as that with the HTL layer, which further confirms the p–n behaviour at the PS/TiO 2 interface. Figure 4: Electrical potential and field profiling results on the optimized planar device. ( a ) Potential profiles taken on the 240-nm device under various V b s. ( b ) Differences or changes between the potentials at the various V b s and V b =0. ( c ) Change in the electric field by V b s. The potential profiles in a are averaged from the potential images along the device lateral direction. The potential changes in b are obtained by subtracting the potential under V b =0 from the potentials under the various V b s. The profiles of the electric field difference in c are deduced by taking a derivative of the potential differences in b . Layer positions are indicated on top of the figure, which are identified from the SEM image shown in Fig. 3a . The potential change in b and the field change in c concentrate around the TiO 2 /PS interface, and decrease towards the HTL, which is consistent with a p–n junction at the interface. Full size image However, the electric field profiles ( Fig. 4c ) exhibit small amplitudes in the HTL and the back-contact layer, which is caused by taking the derivative, because any small imperfection of the potential measurement can be greatly enhanced by this data processing. On the profiles, one also observes ‘waves’ superimposed on the large variation, which results from a smoothening of the potential data before taking the derivative. The smoothening is necessary for obtaining a meaningful field profile; otherwise, any small noise-level change in the potential profile would cause a tremendous change in the field profile. Therefore, we should focus on the large variation of the field profile and omit the small ones. The field profiles exhibit enhanced features compared with the potential profiles. Thick planar device For the thin planar PS device studied above, the potential drop and the nonuniform field extend throughout the whole PS layer. If the PS and n -type TiO 2 /TCO form a p–n junction, then the electric field extension or the junction depletion width depends on the carrier concentration. To determine the depletion width, we fabricated a cell with PS layer thickness of ∼ 1 μm. The profiles of potential, potential change and electric field are displayed in Fig. 5 , and the corresponding AFM and KPFM images at the various V b s are shown in Supplementary Fig. 2 . One observes that the electric field or the potential drop extends ∼ 300 nm from the TiO 2 /PS interface when V b =−1 V, and no field is observed at deeper locations in the PS layer. This further demonstrates the p–n junction structure of the device, and it excludes both the n–i–p junction and the exciton solar cells. 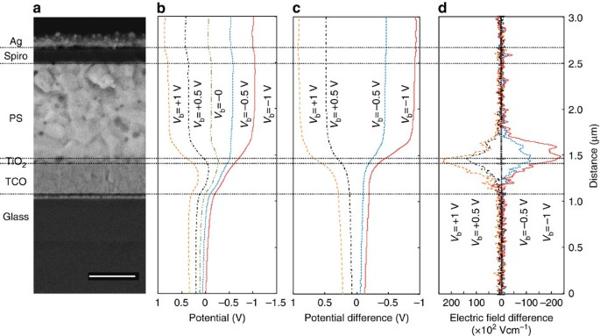Figure 5: Potential profiling and layer structure of the thick planar device. (a) SEM image taken on the cross-section of the 1-μm planar device. (b) Potential profiles under the variousVbs. (c) Potential differences between the potentials at the variousVbs andVb=0. (d) Changes in the electric filed byVbs. Scale bar, 500 nm (a). The potential profiles inbare averaged from the potential images along the device lateral direction. The potential changes incare obtained by subtracting the potential underVb=0 from the potentials under the variousVbs. The profiles of electric field change indare deduced by taking a derivative of the potential differences inc. The layer positions are indicated on the left of the figure, which are identified from the SEM image. The potential change incand the field indconcentrate around the TiO2/PS interface, and decrease towards the HTL, with no field beyond the depletion region of the PS layer. Figure 5: Potential profiling and layer structure of the thick planar device. ( a ) SEM image taken on the cross-section of the 1-μm planar device. ( b ) Potential profiles under the various V b s. ( c ) Potential differences between the potentials at the various V b s and V b =0. ( d ) Changes in the electric filed by V b s. Scale bar, 500 nm ( a ). The potential profiles in b are averaged from the potential images along the device lateral direction. The potential changes in c are obtained by subtracting the potential under V b =0 from the potentials under the various V b s. The profiles of electric field change in d are deduced by taking a derivative of the potential differences in c . The layer positions are indicated on the left of the figure, which are identified from the SEM image. The potential change in c and the field in d concentrate around the TiO 2 /PS interface, and decrease towards the HTL, with no field beyond the depletion region of the PS layer. Full size image The potential profile at V b =0 ( Fig. 5b ) does not reflect the built-in potential in the bulk because of surface charges. Instead of a decreased built-in potential in the device bulk (from TiO 2 towards PS), the profile exhibits a small increase of ∼ 0.2 V, inconsistent with the bulk built-in potential even with an opposite sign. However, we can use the width of surface potential drop ( W ∼ 300 nm) on the profile at V b =−1 V to roughly estimate the depletion width of the p–n junction in the bulk [19] , [20] , because the surface potential drop amplitude at V b =−1 V roughly agrees with the bulk built-in potential V bi ∼ 1.2 V (ref. 13 ). The carrier concentration in the PS layer is roughly estimated to be ∼ 7 × 10 16 cm −3 , using the depletion width W =300 nm, V bi =1.2 V and dielectric constant ɛ =70 (ref. 23 ) This carrier concentration is in the range that is favourable for PV application [4] . Similar to the leading inorganic thin-film solar cells of CdTe and CIGS, there is no intentional foreign doping during the PS film growth and other device fabrication steps. Referring to the intrinsic p -type doping of point defects in CdTe and CIGS, which result from shallow acceptor levels [24] , [25] , we would expect that intrinsic defect doping could be responsible for the p -type carriers in PS film [26] , [27] . However, one report speculates an important role of the HTL layer in the doping of the underlying PS film [13] . To investigate whether the HTL has an effect on the electric field, we measured on a device with identical structure but without the HTL layer, and using a Au back-contact in place of Ag. The potential profiling results are shown in Supplementary Fig. 3 , which demonstrate no effect of the HTL layer on the electric field. There is a trivial topographic effect on the potential imaging. The large particle observed at the top of Supplementary Fig. 2b affects a little the potential imaging in Supplementary Fig. 2c–g . This topographic effect is generally induced by ‘cross-talk’ of the cantilever oscillation at the two frequencies used for the AFM and KPFM imaging. To examine this effect, we draw two example line profiles ( Supplementary Fig. 4 ) that scan across the two large particles in Supplementary Fig. 2b . The potential profiles show a trivial ‘cross-talk’ between AFM and KPFM, as the potential along line 1 ( Supplementary Fig. 4c ) decreases slightly in the region of HTL and Ag, but increases slightly on line 2 ( Supplementary Fig. 4g ). However, the potential changes by V b are identical ( Supplementary Fig. 4d,h ), all showing flat potentials across the device except for the location around the PS/TiO 2 junction. Therefore, there is no observable ‘cross-talk’ in the surface potential change. Although the TCO is grounded, the potential value on the TCO changes with V b ( Figs 4b and 5c ). This change could be attributed to the non-trivial resistance of TCO and partial shunting of the devices created in the cleaving of the device. This current-resistance-induced potential change can also be verified by the larger potential change in TCO with forward V b than reverse V b . It is also noteworthy that the potential profiles on the TCO are not uniform, showing curves in Fig. 5b . This is likely caused by static charges on the cross-sectional surface. The surface can trap significant amount of charges on defects created by cleaving, and the screening of these charges depends on the charge carriers in the surrounding area, which can make the screening length much longer than expected in the TCO bulk. This scenario of the defects and charges can be much different from that of the TCO bulk. Therefore, we must examine the potential change under V b , which can exclude the effect of surface charges as shown in Fig. 5c . Porous device The potential profiling demonstrates that the planar device has a p–n junction at the PS/TiO 2 interface. A question then arises about the fundamental working mechanism of the porous device: do the TiO 2 and porous PS materials also form a similar p–n junction? 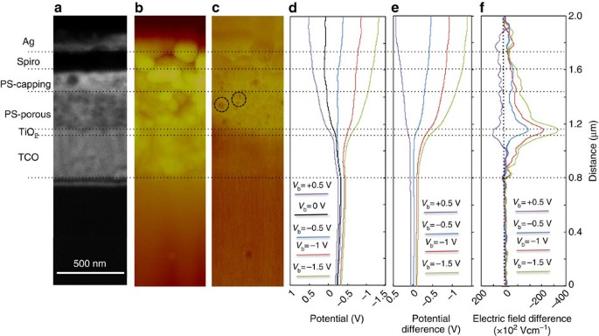Figure 6: Profiles of the electrical potential and field and layer structure of the porous device with optimized thickness. (a) SEM image; (b) AFM and (c) the corresponding KPFM images taken on the cross-section of the 280-nm porous device. (d) Potential profiles under the variousVbs. (e) Potential differences between those with the variousVbs and that withVb=0. (f) Changes in the electric field byVbs. The layer positions are indicated on the left of the figure, which are identified from the SEM image. The electric field covers the TiO2/porous interface and the porous and capping layers, with the maximum at the TiO2/porous interface. Example potential features such as the dark spots indicated by the dashed circles in (c) are caused by charges trapped on the cross-sectional surface. Figure 6 shows the potential profiling results on the porous device with an optimized TiO 2 layer thickness of 280 nm and a PS-capping layer of 160 nm. Because the spatial resolution of KPFM is ∼ 30–50 nm, which is larger or similar to the pore sizes ( ∼ 20–30 nm), the potential image cannot resolve the two components of the TiO 2 and the PS networks in the porous layer. The features in Fig. 6c , such as indicated by the circles, correspond to surface charges rather than the potential contrasts of the two components. If the features arose from the contrast of the components, one would expect a change in the contrast with V b . However, if it is induced by surface charges, the contrast should not change with V b , which is the case as shown in the potential images of Supplementary Fig. 5 . Therefore, the average along the lateral direction does not sacrifice the potential fine features. The average excludes the effect of local artefacts and enhances the signal/noise ratio, as in the case of planar devices. The electric field in this device covers mainly the TiO 2 /porous-PS interface, porous-PS layer and PS-capping layer ( Fig. 6f ). The electric field in the porous and capping layers overlaps at the porous/capping interface. The small electric field in the HTL and back-contact are due to insignificant imperfection of the measurement. KPFM utilizes two separate frequencies to probe surface morphology and potential, respectively. In general, these two measurements cannot be completely decoupled even with low- and high-pass filters. Thus, surface corrugation can be convoluted (insignificantly) with the potential signal. Therefore, we should focus on the large bias-voltage-induced potential features, which reflect the potential in the bulk across the device. Figure 6: Profiles of the electrical potential and field and layer structure of the porous device with optimized thickness. ( a ) SEM image; ( b ) AFM and ( c ) the corresponding KPFM images taken on the cross-section of the 280-nm porous device. ( d ) Potential profiles under the various V b s. ( e ) Potential differences between those with the various V b s and that with V b =0. ( f ) Changes in the electric field by V b s. The layer positions are indicated on the left of the figure, which are identified from the SEM image. The electric field covers the TiO 2 /porous interface and the porous and capping layers, with the maximum at the TiO 2 /porous interface. Example potential features such as the dark spots indicated by the dashed circles in ( c ) are caused by charges trapped on the cross-sectional surface. Full size image To determine how deep the electric field extends into the porous layer, we fabricated a device with a porous layer thickness of 850 nm and a capping layer thickness of 130 nm. The results ( Fig. 7 ) show that the electric field covers the interface and layers, similar to the thin device, with the electric field covering the full range of the thick porous layer. The corresponding potential images under various V b s are shown in Supplementary Fig. 6 . This distribution of the electric field is different from the thick planar device, where no electric field is observed beyond the depletion region. The amplitude of the electric field or the potential drop in the thick porous PS device decreases in the order of TiO 2 /porous-interface>PS-capping>porous layer. 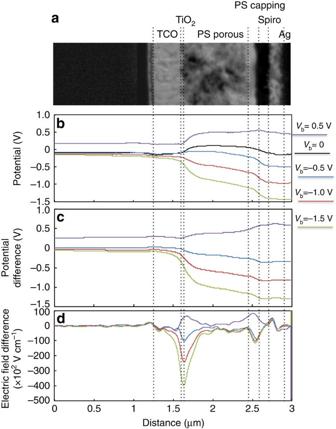Figure 7: Layer structure and potential/field profiles of the thick porous device. (a) An SEM image taken on the cross-section of the 850-nm porous device. (b) Potential profiles under the variousVbs, as averaged from the potential images. (c) Potential differences between the profiles under the variousVbs and underVb=0. (d) Changes in the electric field byVbs. The layer positions are indicated on the top of the figure, which are identified from the SEM image. The potential drop and the electric field cover the TiO2/porous interface, the full range of the thick porous layer and the capping layer. Figure 7: Layer structure and potential/field profiles of the thick porous device. ( a ) An SEM image taken on the cross-section of the 850-nm porous device. ( b ) Potential profiles under the various V b s, as averaged from the potential images. ( c ) Potential differences between the profiles under the various V b s and under V b =0. ( d ) Changes in the electric field by V b s. The layer positions are indicated on the top of the figure, which are identified from the SEM image. The potential drop and the electric field cover the TiO 2 /porous interface, the full range of the thick porous layer and the capping layer. Full size image These results on the porous devices are consistent with p–n junctions at PS/TiO 2 interfaces. Similar to the p–n junction in the planar device, the dominant potential drop at the TiO 2 /porous interface indicates a junction at this interface that plays a dominant role in device operation. Different from the planar device, however, the potential drop at the porous and porous/capping interfaces is also significant. This distribution of potential/field across the device implies an n–p − junction at the TiO 2 /porous interface, a weakly doped p − -porous layer and a p − /p potential barrier at the porous/capping interface. The effective p − doping concentration of the porous layer is expected to be relatively low, so that the field extends across the entire porous layer. Because of the small sizes ( ∼ 20–30 nm) for both TiO 2 and PS in the nanoporous layer, the mixture of TiO 2 and PS can be viewed as a distributed heterointerface structure. This type of blend structure can be described by a homogeneous, effective medium [28] , where the one-dimensional macroscopic electric field along the film thickness is important to charge transport. The weak p − -doping of the porous layer is presumably caused by n -type TiO 2 compensating partially p -type PS. The p − /p potential barrier at the porous/capping interface can reflect minority carrier (electrons), and thus is beneficial for carrier collection. This is similar to a back surface field as often used in an inorganic solar cell [29] . The potential profiling results demonstrate that a p–n junction is formed in the PS devices, similar to polycrystalline CdTe and CIGS solar cells [5] . However, unlike inorganic cells, in which the dominant carrier-transport mechanism is diffusion [5] , we infer drift transport in the PS devices, by combining the potential data with the solar cell performance parameters of devices, based on both the relatively thin and thick PS films. The depletion width of the planar device ( ∼ 300 nm) is consistent with the PS film thickness normally reported with good device efficiencies. This indicates that a field is needed for efficient carrier collection. This is consistent with often-observed relatively poor fill factor (FF) (for example, FF=69.6%; Table 1 ) compared with standard high-performance CIGS and CdTe (FF ∼ 80%) [4] . Therefore, the minority-carrier diffusion length in this study is likely to be significantly shorter than that in the inorganic materials ( ∼ 1 μm) [5] . This limitation could be attributed to carrier mobility and/or minority-carrier lifetime. From the high open-circuit voltage ( V oc ) of the 240-nm device ( Table 1 ), we would expect a decent minority-carrier lifetime [9] . Therefore, the carrier mobility is likely to be responsible for the poor diffusion length, because the diffusion length L d related with the minority-carrier lifetime τ e and mobility μ : L d =sqrt (τ e μkTq −1 ), where k , T and q are Boltzmann constant, temperature and elementary change, respectively. Indeed, series resistance ( R s ) of the optimized device, R s ∼ 5 Ω cm 2 ( Table 1 ), is significantly larger than that of the high-performance CdTe and CIGS cells ( R s <1 Ω cm 2 ). This R s value lowers the voltage output by ∼ 100 mV at the maximum power output point; hence reducing the FF by ∼ 10%. Although a mobility of 8 cm 2 V − 1 s − 1 (ref. 10 ) of CH 3 NH 3 PbI 3 PS is a good value compared with most solution-processed organic PV materials, it is one or two orders of magnitude lower than the leading inorganic materials [5] , which could be the reason for the shorter diffusion length in comparison with that in inorganic materials. It is worth noting that for a planar PS thin film ( ∼ 270 nm) a diffusion length of the order of 1 μm has been reported [9] . However, at this film thickness, the PS grain could span the entire thickness of the film (for example, Fig. 3a ), and thus the GBs will not likely play a significant role in charge transport across the thickness of the PS layer. When the film thickness is increased substantially (for example, ∼ 1 μm), the large number of GBs (for example, Fig. 5a ) will likely scatter transport across the thickness of the film, leading to reduced diffusion length in thicker films. A recent study shows that the optimum device architecture depends on the diffusion length, mobility-lifetime product of the absorber layer and their relationship with the absorber layer thickness [30] . To obtain such information, more fundamental studies are required in the future to verify the discussions above. As the planar PS thickness increases to 1 μm, FF is the most affected among the performance parameters ( Table 1 ), which is consistent with the poor diffusion length. The SEM image taken on the cross-section of the 240-nm device ( Fig. 3a ) indicates a single layer of PS grains; the image on the 1-μm device ( Fig. 5a ) suggests multiple grains in the device vertical direction. Therefore, scattering at GBs could be a contributing factor to the poor diffusion length, which is consistent with the discussion above. Developing PS films with a single layer of grains with different film thickness will help to elucidate the effect of the GBs on charge transport across the PS layer. Finally, we compare the PS device with the record CdTe thin-film cell ( E ff =21.0%) [4] , with only small differences in the bandgap (PS is 1.55 eV, CdTe is 1.45 eV). Our PS cell has a higher V oc (1.07 versus 0.88 V), a lower short-circuit current density ( J sc =21.6 versus 30.3 mA cm − 2 ), and lower FF (69.6 versus 79.4%). The high V oc indicates a proper carrier concentration and good junction quality. Since the bandgap difference of ∼ 0.1 eV at the bandgap of ∼ 1.5 eV should ideally lead to a J sc difference of ∼ 4 mA cm − 2 (ref. 31 ), the observed substantially lower J sc value indicates inadequate light absorption, which is attributable to the thin absorber layer. Although PS absorbs light strongly, its absorption at the long wavelength range near the absorption edge ( ∼ 800 nm) is less ideal. This is also reflected from the external quantum efficiency spectra ( Supplementary Fig. 7 ) for a thin ( ∼ 250 nm) planar device. It is clear that external quantum efficiency drops quickly at wavelength longer than 650 nm, suggesting that thicker PS films are needed for further improving J s c . The low FF can be ascribed to the nonideal field-assisted carrier collection associated with the poor carrier mobility. J sc should be improved by increasing the PS thickness. If the diffusion length and mobility in the PS material can be improved, a higher FF value in a thickened PS device is expected. In summary, we have studied the carrier separation and transport in PS solar cells—the fundamental mechanisms of device operation—by determining the junction structure across the devices. We found that the electric field in the planar TiO 2 /PS device concentrates around the TiO 2 /PS interface with a depletion width of ∼ 300 nm. This demonstrates the p–n junction structure and the minority-carrier diffusion/drift operation of the devices, rather than the mechanism of exciton separation at the interface. The electric field in the porous device covers the TiO 2 -layer/porous-PS interface, and the porous-PS and PS-capping layers, with amplitudes in the decreasing order of TiO 2 /PS-interface>PS-capping>porous-PS. This distribution of electric field is also consistent with the p–n junction at PS/TiO 2 interfaces in the device. Our results suggest that for thicker PS films the carrier mobility may be the limiting factor that needs to be improved for further improving device efficiency. Device fabrication Fluorine-doped tin oxide (FTO) substrates (TEC15, Hartford, USA) were cleaned by immersing in a base bath (5 wt% NaOH ethanol solution) overnight, and rinsed thoroughly with deionized water and ethanol. A thin compact TiO 2 layer was deposited on top of FTO by spray pyrolysis using 0.2 M Ti(IV) diisopropoxide bis(acetylacetonate) in 1-butanol solution at 450 °C. For mesoporous structure, 280-nm and 850-nm TiO 2 layers were printed using a screen printer by controlling emulsion thickness of the screens. PS film was prepared by adapting procedures from previous reports [32] , [33] , [34] . Briefly, planar samples (240 and 1,000 nm) were prepared through spin-coating 42 and 60 wt% of stoichiometric lead iodide (PbI 2 ) and methylammonium iodide in 1-methyl-2-pyrrolidinone/γ-butyrolactone (7/3, weight ratio) solution at 4,500 r.p.m. for 15 s. These films were then transferred into a diethyl ether bath for 2 min, followed by a heating at 150 °C for 2 min. For preparing mesoporous samples, the precursor was made of ∼ 44 wt% of 1:1 molar ratio of methylammonium iodide and PbI 2 in γ-butyrolactone/dimethyl sulfoxide (7/3 v/v). Substrates with different mesoporous layers (280 nm, 850 nm) were spin-coated at 4,500 r.p.m. for 50 s, and a drop of toluene was dripped during the spinning process. These films were then annealed at 85 °C for 10 min. The thickness of the PS film was controlled by changing precursor concentration (40–60 wt%) and spin-coating speed (2,000–5,000 r.p.m.). Then, a HTL was cast on top of the PS film by spin-coating a spiro-OMeTAD solution at 3,000 r.p.m. for 30 s. The spiro-OMeTAD solution is composed of 80 mg 2,2′,7,7′-tetrakis( N , N -dip-methoxyphenylamine)-9,9′-spirobifluorene (spiro-MeOTAD), 30 μl bis(trifluoromethane)sulfonimide lithium salt stocking solution (500 mg Li-TFSI in 1 ml acetonitrile), 30 μl 4-tert-butylpyridine and 1 ml chlorobenzene solvent. Finally, a 150-nm silver film was deposited on top of HTL by a thermal evaporator using a shallow mask. KPFM characterization The PS devices were cleaved to expose the cross-section for potential profiling across the device. In brief, we first make a notch on the device side in areas outside the device boundary, and then cleave the device from the device side (not from the glass-substrate side), so that the device was cleaved by tension rather than by compression. In this way, the cross-section of the PS device is often adequately flat for AFM and KPFM measurements. KPFM was employed for the potential imaging, which measures the contact potential difference between the probe (Nanosensor PPP-EFM) and sample by detecting the alternating current–voltage-induced AFM cantilever oscillation using a wide-bandwidth and low-noise lock-in amplifier (Signal Recovery 7,208). A negative-feedback analogue circuit using the cantilever oscillation signal (the lock-in amplifier output) as a feedback source generates the contact potential difference or Kelvin probe signal, which also constantly nullifies the cantilever oscillation. The workfunction of the probe remains unchanged during the AFM scanning. The sum of Kelvin probe voltage and alternating current–voltage (1 V) is applied to the probe. The image of the Kelvin probe signal represents the relative scale of the electrostatic potential on the sample surface. In our set-up, the first resonant oscillation of the cantilever (50–70 kHz) was used for the non-contact AFM (Veeco D5000 and Nanoscope V) topographic imaging. The second resonant frequency (300–500 kHz) was used for the potential imaging, which gives an enhanced energy resolution of ∼ 10 mV in the atmospheric pressure, compared with the conventional set-up using a low frequency of ∼ 20 kHz ( ∼ 50 mV). The scan rate is 0.2 Hz. The FTO layer of the device is grounded. V b is applied to the device through the metal back-contact of the superstrate devices. When a bias voltage ( V b ) is applied to the device with extended amplitude and duration, the bias voltage may induce significant ion migration [35] , [36] , which can complicate the results of potential profiling. To avoid this complication, we first took the potential profiling at V b =0, and then applied V b step by step in a small voltage interval (for example, 0.5 V) and short time interval (for example, 5 min). Then, the potential at V b =0 was retaken to check no change in the potential image. The maximum reverse V b was –1.5 V. The maximum forward V b was +0.75 V on the optimized (and +1 V on the thickened) devices. We found no significant effect of ion migration under these conditions. This is supported by having no changes of the potential line profiles during the 5-min scanning and also by having consistent change in electric field when changing V b . It is worth noting that the effect of ion migration under extended bias voltage amplitude and duration is expected to affect the potential profiling, and this will be a subject of future study. In addition, we have ensured no significant illumination effect on the potential profiling results. The measurement was carried out in the dark. However, there is a weak unintentional illumination of the AFM laser (1.8 eV and 100 μm in diameter). The cantilever width is 40 μm, which blocks the laser illumination on the area right beneath the probe tip. In this case, there is some leaking of light in areas of about 20 μm away from the area that is probed by KPFM. This distance is much larger than film thickness of the device. To be certain, we have also used a cantilever with a hammerhead shape, which blocks the entire AFM laser by the 100-μm-wide cantilever. The results are consistent with that using the normal KPFM probe. Device characterization The current density–voltage (J–V) curves were measured by a source meter (Keithley 2400) under AM 1.5G illumination (Oriel Sol3A class AAA solar simulator) at a scan rate of 20 mV s − 1 . A typical active area of 0.12 cm 2 was defined using a non-reflective mask for the J–V measurements. J–V curves with both forward and reverse scans taken on the four devices are shown in supplementary Fig. 8 , and the solar cell performance parameters obtained from the J – V curves are listed in supplementary Table 1 . How to cite this article: Jiang, C.-S. et al . Carrier separation and transport in perovskite solar cells studied by nanometre-scale profiling of electrical potential. Nat. Commun. 6:8397 doi: 10.1038/ncomms9397 (2015).